An RNA-seq method for defining endoribonuclease cleavage specificity identifies dual rRNA substrates for toxin MazF-mt3 Toxin–antitoxin (TA) systems are widespread in prokaryotes. Among these, the mazEF TA system encodes an endoribonucleolytic toxin, MazF, that inhibits growth by sequence-specific cleavage of single-stranded RNA. Defining the physiological targets of a MazF toxin first requires the identification of its cleavage specificity, yet the current toolkit is antiquated and limited. We describe a rapid genome-scale approach, MORE (mapping by overexpression of an RNase in Escherichia coli ) RNA-seq, for defining the cleavage specificity of endoribonucleolytic toxins. Application of MORE RNA-seq to MazF-mt3 from Mycobacterium tuberculosis reveals two critical ribosomal targets—the essential, evolutionarily conserved helix/loop 70 of 23S rRNA and the anti-Shine-Dalgarno (aSD) sequence of 16S rRNA. Our findings support an emerging model where both ribosomal and messenger RNAs are principal targets of MazF toxins and suggest that, as in E. coli , removal of the aSD sequence by a MazF toxin modifies ribosomes to selectively translate leaderless mRNAs in M. tuberculosis . Toxin–antitoxin (TA) systems comprise tandem, co-regulated genes encoding a stable toxin and a relatively unstable antitoxin. TA systems are ubiquitous in free-living prokaryotes and are the subject of intense interest because they are abundant in bacterial pathogens and implicated in stress survival, virulence and persistence [1] , [2] , [3] . One of the best characterized TA modules is mazEF , an operon in Escherichia coli that encodes the intracellular toxin MazF and its cognate inhibitor, antitoxin MazE. During unstressed conditions, the MazE protein forms a stable complex with MazF to neutralize its toxicity [4] . However, upon encountering stresses such as nutrient limitation [4] , [5] , MazE is degraded, liberating the MazF toxin, a single-strand and sequence-specific endoribonuclease [6] , [7] . Growth arrest mediated by MazF in E. coli is characterized by a state of suspended animation in which cells appear to retain the capacity to resume full metabolic activity [8] . Thus, E. coli MazF appears to facilitate cell survival during relatively short periods of stress [9] . The dynamic exchange between the free toxin in an active state and the inactive antitoxin-bound state underlies the reversibility of toxin-mediated growth arrest. If, however, the free MazF toxin is not disabled by subsequent expression of MazE before a ‘point of no return,’ E. coli MazF triggers bacterial cell death [10] . Mycobacterium tuberculosis is a pathogen that contains an unusual abundance of TA systems (>80 putative TA pairs) [11] , including nine MazF orthologs. In contrast to E. coli , the physiological roles of TA systems in M. tuberculosis are not known, nor is it understood why there are so many seemingly redundant genes. The striking similarities between the state of ‘quasi-dormancy’ induced by MazF in E. coli [8] and the nonreplicating persistent state of M. tuberculosis during latent infection raise the possibility that these nine MazF orthologs play a role in M. tuberculosis persistence and dormancy [1] , [2] , [3] . The effects of MazF toxins on cellular growth have been proposed to occur as a consequence of the specific targeting of mRNAs [6] , [7] , [12] , [13] , [14] , [15] , [16] , [17] , [18] , [19] , [20] , [21] . According to this ‘mRNA interferase’ model, cleavage target sequences embedded within transfer RNA (tRNA) and rRNA are refractory to the action of MazF toxins [7] , [8] , [12] , [13] , [16] , [17] , because these RNAs contain extensive regions of secondary structure and, in the case of rRNA, interactions with ribosomal proteins. However, the view that MazF toxins act exclusively by targeting mRNA has been challenged by recent studies demonstrating that E. coli MazF cleaves 16S rRNA [22] and that the M. tuberculosis ortholog MazF-mt6 cleaves 23S rRNA [23] . All MazF orthologs characterized to date cleave single-stranded RNA at specific 3-, 5- or 7-nt recognition sequences, nearly all of which are unique [7] , [14] , [15] , [16] , [17] , [18] , [19] , [20] , [21] , [23] , [24] , [25] , [26] . Because each MazF toxin requires a strict RNA recognition sequence for cleavage, one cannot predict the physiological targets of a given MazF ortholog without first determining its distinct cleavage specificity. Standard methods for defining the cleavage recognition sequence primarily involve: primer extension analysis of RNA harvested from cells in which the endoribonuclease is ectopically expressed [6] , [7] , [16] , [17] , [18] , [21] , [23] , [24] , [25] , [26] , [27] , [28] ; primer extension analysis of substrate RNAs incubated with recombinant enzyme in vitro [14] , [15] , [16] , [19] , [20] , [24] , [25] , [26] , [28] , [29] ; or analysis of cleavage products generated from short RNA oligonucleotides incubated with recombinant enzyme in vitro [6] , [7] , [15] , [16] , [17] , [18] , [21] , [26] . These methods often lead to reports of inaccurate or ambiguous cleavage recognition sequences [14] , [17] , [18] , [20] , [21] , [27] , [28] , [29] or discrepancies in the position of cleavage [6] , [7] , [17] , [21] , [23] , [24] , [25] , [27] , [29] . In addition, use of conventional methods to identify relatively long recognition sequences (>4-nt) is, at best, time-intensive [16] and, at worst, impossible if the recognition sequence is underrepresented in the collection of substrate RNAs that are analysed. Here we describe an alternative methodology to derive cleavage consensus sequences for endoribonuclease toxins that would overcome the inherent limitations of conventional approaches. Our approach, which we term MORE (mapping by overexpression of an RNase in E. coli ) RNA-seq, involves ectopic production of the toxin in E. coli , selective enrichment of RNAs generated upon toxin cleavage and cleavage site identification using RNA-seq. Using MORE RNA-seq, we define the cleavage specificity of one of the nine MazF orthologs in M. tuberculosis , MazF-mt3 (locus Rv1991c ). In contrast to conventional approaches, MORE RNA-seq identifies an unambiguous cleavage recognition sequence (UCCUU), precisely maps the position of cleavage within this sequence (U↓CCUU, where ‘↓’ indicates the position of cleavage) and allows a determination of whether the ends generated upon cleavage carry a 5′-hydroxyl or a 5′-monophosphate (5′-hydroxyl in the case of MazF-mt3). Among the MazF-mt3 cleavage sites identified in the E. coli transcriptome by MORE RNA-seq are two sites within the critical positions of 23S and 16S rRNA that are conserved in M. tuberculosis . Remarkably, in spite of recognizing a distinct sequence, MazF-mt3 cleaves 23S rRNA within the helix/loop 70 at the same position as M. tuberculosis MazF-mt6 (ref. 23 ). MazF-mt3 also cleaves within the anti-Shine-Dalgarno (aSD) sequence at the 3′ end of 16S rRNA. In contrast, only 20% of M. tuberculosis mRNAs are predicted to be susceptible to cleavage by MazF-mt3. Our findings support an emerging model in which both rRNA and mRNA serve as prominent targets of M. tuberculosis MazF toxins. An RNA-seq approach to determine toxin cleavage specificity We sought to develop a generally applicable high-throughput approach to derive cleavage consensus sequences for endoribonuclease toxins that would overcome the inherent limitations of conventional approaches. We reasoned that the use of an RNA-seq-based approach would save time and increase accuracy by providing base-pair resolution and by enabling the analysis of hundreds of substrate RNAs in parallel. Thus, our strategy was to ectopically produce an endoribonuclease in E. coli , identify cleavage sites in the transcriptome using a modified form of RNA-seq and derive a consensus sequence by aligning the cleavage sites. E. coli represents a valuable surrogate to identify cleavage sites for two reasons. First, E. coli is highly genetically tractable. Many extremophilic, fastidious or pathogenic organisms, however, contain high numbers of uncharacterized endoribonucleolytic toxins, and genetic tools for manipulation of these organisms are very limited or absent. In addition, these organisms typically require specialized conditions to grow in the laboratory. These drawbacks make it infeasible to characterize the toxins they carry in their native context. Second, E. coli , unlike many of the organisms containing uncharacterized endoribonucleolytic toxins, does not contain a 5′-to-3′ exoribonuclease. Thus, the 5′ ends generated upon endoribonuclease cleavage will not subsequently be processed as they would in the native context. Therefore, cleavage sites in E. coli can be readily identified as RNA 5′ ends that are present in cells containing the endoribonuclease and absent in cells that do not. To validate the utility of this approach, we determined the cleavage recognition sequence of the toxin MazF-mt3 from the bacterial pathogen M. tuberculosis . Identifying the cleavage specificities for the large number of uncharacterized endoribonucleolytic toxins from M. tuberculosis [11] is particularly challenging in their native context because M. tuberculosis is slow growing (doubling every 24 h), requires BSL3 containment, and lacks experimental tools for detailed molecular manipulation. In addition, M. tuberculosis contains at least one 5′-to-3′ exoribonuclease (RNase J, locus Rv2752 ) [30] . We chose MazF-mt3 for our initial analysis because the cleavage specificity of this endoribonuclease had previously been analysed by a conventional approach and was proposed to require a degenerate 5-nt sequence (CU↓CCU or UU↓CCU; where↓indicates the position of cleavage) [20] . Thus, we could directly compare the results from our high-throughput approach with conventional approaches. Consistent with prior studies [21] , growth of E. coli cells was arrested after the initiation of MazF-mt3 toxin production. This MazF-mt3-induced growth arrest was reversible, since subsequent expression of antitoxin MazE-mt3 restored growth ( Supplementary Fig. 1 ). For our RNA-seq-based approach, we introduced either a vector that directs the synthesis of MazF-mt3 under the control of an arabinose-inducible promoter or an empty plasmid into E. coli , grew cells to mid-exponential phase and added arabinose to the growth medium to initiate MazF-mt3 production. To identify MazF-mt3-dependent cleavage sites, we harvested total RNA at a time coinciding with the commencement of growth arrest in MazF-mt3-carrying cells (that is, 15 min after the addition of arabinose). We then analysed these RNAs using a modified form of RNA-seq that examines cDNAs derived only from RNAs possessing one of two types of 5′ ends potentially generated after endonucleolytic cleavage—a 5′-monophosphate (5′-P) or a 5′-hydroxyl (5′-OH). Although the four MazF toxins characterized to date [6] , [18] , [29] , [31] produce an RNA fragment with a 5′-OH ( Fig. 1a ), this mode of cleavage has not been formally demonstrated for MazF-mt3. Therefore, the 5′-ends generated upon MazF-mt3-dependent cleavage could either carry a hydroxyl or a monophosphate. To distinguish between these two possibilities, we employed a cDNA library construction protocol that isolates transcripts based on their 5′-end phosphorylation status ( Fig. 1b ). Thus, the protocol can be tailored such that cDNAs are generated only from transcripts carrying a 5′-OH or only those transcripts carrying a 5′-P. 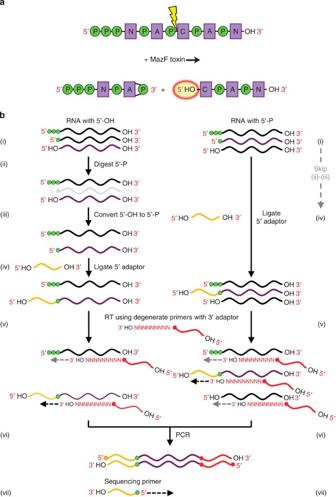Figure 1: MORE RNA-seq cDNA library construction. (a) Cleavage of RNA with MazF toxins yields two fragments—one with a 2′,3′-cyclic phosphate and one with a 5′-hydroxyl. P, phosphate; N, A, C, nucleosides; OH, hydroxyl. (b) Procedures for generating cDNA libraries derived from RNAs carrying only a 5′ hydroxyl (5′-OH) or only a 5′ monophosphate (5′-P). (i) Depicted are RNAs with a 5′ triphosphate, a 5′-P, or a 5′-OH; the species that will be converted into cDNA is shown in purple, and phosphate groups are depicted by green circles. Steps (ii) and (iii) are specific to generation of cDNAs from 5′-OH. (ii) RNAs with a 5′-P are removed by treatment with a 5′-P-specific exonuclease. (iii) RNA with a 5′-OH is phosphorylated by a kinase. (iv) The 5′ adaptor is ligated to RNAs that carry a 5′-P. (v) Reverse transcription (RT) using a primer with a 9-nt degenerate sequence at the 3′ end and the sequence of the 3′ adaptor at the 5′ end. (vi) PCR amplification using primers that match the 5′ and 3′ adaptors (only cDNAs that contain both 5′ and 3′ adaptor sequences can be amplified). (vii) The SOLiD sequencing ligation reaction originates from a primer complementary to the 5′ adaptor. The first base of each sequencing read corresponds to the 5′ end of an RNA transcript. Figure 1: MORE RNA-seq cDNA library construction. ( a ) Cleavage of RNA with MazF toxins yields two fragments—one with a 2′,3′-cyclic phosphate and one with a 5′-hydroxyl. P, phosphate; N, A, C, nucleosides; OH, hydroxyl. ( b ) Procedures for generating cDNA libraries derived from RNAs carrying only a 5′ hydroxyl (5′-OH) or only a 5′ monophosphate (5′-P). (i) Depicted are RNAs with a 5′ triphosphate, a 5′-P, or a 5′-OH; the species that will be converted into cDNA is shown in purple, and phosphate groups are depicted by green circles. Steps (ii) and (iii) are specific to generation of cDNAs from 5′-OH. (ii) RNAs with a 5′-P are removed by treatment with a 5′-P-specific exonuclease. (iii) RNA with a 5′-OH is phosphorylated by a kinase. (iv) The 5′ adaptor is ligated to RNAs that carry a 5′-P. (v) Reverse transcription (RT) using a primer with a 9-nt degenerate sequence at the 3′ end and the sequence of the 3′ adaptor at the 5′ end. (vi) PCR amplification using primers that match the 5′ and 3′ adaptors (only cDNAs that contain both 5′ and 3′ adaptor sequences can be amplified). (vii) The SOLiD sequencing ligation reaction originates from a primer complementary to the 5′ adaptor. The first base of each sequencing read corresponds to the 5′ end of an RNA transcript. Full size image We prepared 5′-OH and 5′-P cDNA libraries using total RNA isolated from biological replicates of cells that did or did not contain MazF-mt3. These cDNA libraries were sequenced using a SOLiD (sequence by oligonucleotide ligation and detection) Analyzer. For each sample, we obtained between 12 and 23 million sequencing reads that aligned to the E. coli genome with no mismatches ( Supplementary Table 1 ). The first base of each individual sequencing read corresponds to the first base of the 5′ end of an RNA. Thus, to identify 5′ ends derived from cleavage, we first determined a value for each position in the genome that we term ‘#5′-ends.’ For any given position in the genome, the #5′-ends correspond to the total number of sequencing reads whose first base aligns to this position. We then identified genomic positions for which the #5′-ends observed in the cells containing MazF-mt3 were at least 50-fold higher than in the cells that did not contain MazF-mt3. While analysis of the sequencing reads derived from 5′-P ends identified only two genomic positions that met this criterion, comparison of the reads derived from 5′-OH ends identified 273 such positions ( Supplementary Data 1 ). For the purpose of illustration, Fig. 2a,b shows the identification of four of the 273 positions of enrichment. One of these positions was within talB (transaldolase B; Fig. 2a,b ) while three others were within glpA (anaerobic glycerol-3-phosphate dehydrogenase, subunit A; Fig. 2a,b ). 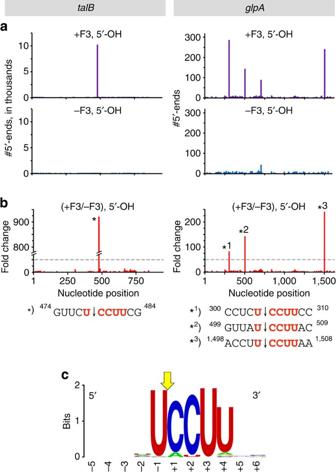Figure 2: Determination of the MazF-mt3 cleavage recognition sequence by MORE RNA-seq. (a) Histograms representing the #5′-ends observed intalB(left) andglpA(right) from the analysis of RNAs carrying a 5′-OH isolated from cells containing MazF-mt3 (+F3) or cells without MazF-mt3 (−F3). (b) Histogram representing the ratio of the #5′-ends observed in cells containing MazF-mt3 versus the #5′-ends in cells that did not contain MazF-mt3. The ≥50-fold increase cutoff is marked with a dotted grey line. RNA sequences surrounding the indicated cleavage sites (labelled with an asterisk (*) in the histograms) are shown below. (c) Sequence logo55generated by aligning the RNA sequences surrounding the 273 sites for which the #5′-ends with a 5′-OH was ≥50-fold higher in cells containing MazF-mt3 than in cells that did not contain MazF-mt3 (Supplementary Data 1). The numbering reflects the nucleotide position relative to the exact point of cleavage, indicated by the yellow arrow. Figure 2: Determination of the MazF-mt3 cleavage recognition sequence by MORE RNA-seq. ( a ) Histograms representing the #5′-ends observed in talB (left) and glpA (right) from the analysis of RNAs carrying a 5′-OH isolated from cells containing MazF-mt3 (+F3) or cells without MazF-mt3 (−F3). ( b ) Histogram representing the ratio of the #5′-ends observed in cells containing MazF-mt3 versus the #5′-ends in cells that did not contain MazF-mt3. The ≥50-fold increase cutoff is marked with a dotted grey line. RNA sequences surrounding the indicated cleavage sites (labelled with an asterisk (*) in the histograms) are shown below. ( c ) Sequence logo [55] generated by aligning the RNA sequences surrounding the 273 sites for which the #5′-ends with a 5′-OH was ≥50-fold higher in cells containing MazF-mt3 than in cells that did not contain MazF-mt3 ( Supplementary Data 1 ). The numbering reflects the nucleotide position relative to the exact point of cleavage, indicated by the yellow arrow. Full size image Alignment of the genomic sequences five bases up- and downstream of the 273 positions of enrichment revealed a strong 5-base consensus sequence, UCCUU, from −1 to +4, where +1 is the position of enrichment ( Fig. 2c ). The convergence of these 273 positions on a clear consensus sequence indicates that most, if not all, of these positions represent MazF-mt3 cleavage sites. Thus, our findings establish that the MazF-mt3 recognition sequence is U↓CCUU, where ‘↓’ is the position of cleavage. Among the 273 cleavage sites we identified ( Supplementary Data 1) , 80% (219 of 273) were an exact match to the consensus (including the sites within talB and glpA , Fig. 2b ) and 98% (267 of 273) match at four out of five positions. Furthermore, because we identified 273 sites that converged on a clear consensus sequence in the analysis of 5′-OH ends ( Supplementary Data 1 ) and only two sites with no sequence similarity in the analysis of 5′-P ends, we further conclude that MazF-mt3 generates 5′-OH ends upon cleavage. MazF-mt3 cleaves several M. tuberculosis mRNAs Having identified the cleavage recognition sequence for MazF-mt3, we next sought to gain insight into its physiological function in M. tuberculosis by identifying potential targets. We first performed a statistical analysis to determine which M. tuberculosis RNAs might be resistant or susceptible to MazF-mt3 cleavage. To do this, we compared the probability of the expected occurrence of UCCUU within each gene to the actual occurrence. First, we determined that 80% (3,283 of 4,095) of M. tuberculosis ORFs and non-coding RNAs lack the UCCUU cleavage motif and were predicted to be resistant to MazF-mt3 cleavage. Second, we found that 14 genes have a statistically significant ( P -value by binomial test ≤0.05) overrepresentation of the cleavage motif ( Supplementary Table 2 ), suggesting these genes might be preferentially targeted by MazF-mt3. It is well established that transcripts lacking a given recognition motif are stable in the presence of MazF toxins [16] , [19] , [25] and that there is a direct correlation between the number of motifs within a given transcript and its susceptibility to degradation [19] , [25] . To test whether any of the M. tuberculosis genes predicted to be preferred MazF-mt3 targets are indeed cleaved by the toxin, we treated M. tuberculosis total RNA with purified MazF-mt3 and performed RT–PCR analysis of the two transcripts predicted to be most susceptible to MazF-mt3 cleavage ( Supplementary Table 2 ), Rv1685c ( Fig. 3a ) and Rv1545 ( Fig. 3b ). We also analysed tuf (translation elongation factor, thermal unstable; Fig. 3c ), a gene with no MazF-mt3 motifs, and senX3 (sensor-like histidine kinase; Fig. 3d ), a gene whose 5′ UTR contains a single UCCUU motif but whose ORF has none. After treatment with MazF-mt3, regions in the Rv1685c ( Fig. 3e ) or Rv1545 ORFs ( Fig. 3f ) or in the senX3 5′ UTR ( Fig. 3h ) that contain one to four UCCUU motifs no longer generated an amplified product, indicating that these regions had been cleaved by MazF-mt3 (see Supplementary Fig. 2 for complete gel images). In contrast, regions in the tuf ( Fig. 3g ) and senX3 ORFs ( Fig. 3i ) that contain no UCCUU motifs generated equivalent amplicons both in the absence (lane 3) and presence (lane 5) of MazF-mt3. 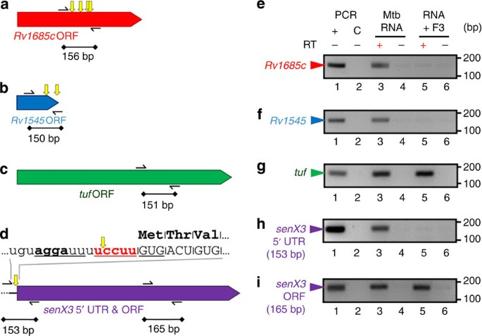Figure 3:MazF-mt3 cleaves severalM. tuberculosismRNAs. Scale schematics ofM. tuberculosisgenes that contain either two or more MazF-mt3 UCCUU motifs (a,b), no MazF-mt3 motifs (c) or one UCCUU motif in the 5′ UTR but none in the ORF (d). Thin black arrows correspond to primers used for RT–PCR, while black lines with diamonds correspond to regions amplified by RT–PCR. Yellow arrows above genes show the location of UCCUU motifs. (d) Text above the schematic represents the RNA sequence of thesenX35′ UTR (lowercase) and ORF (uppercase), with the lone MazF-mt3 motif in bold red text and a putative SD sequence in bold text. (e–i) RT–PCR ofM. tuberculosistotal RNA incubated with (lanes 5 and 6) or without (lanes 3 and 4) purified MazF-mt3 and with (lanes 3 and 5) or without reverse transcriptase (RT; lanes 1, 2, 4 and 6). ‘PCR +’ indicates amplification using the appropriate PCR fragment as a template (lane 1), while ‘C’ is a negative control with H2O as a PCR template (lane 2). Length of DNA size marker in bp is noted by tick marks on the right. After treatment with MazF-mt3, regions that contain one or more UCCUU motifs (e,f,h) no longer generated amplified products. This MazF-mt3-mediated cleavage was specific to regions containing one or more UCCUU motifs, since the amplified products intuf(g) and in thesenX3ORF (i) were comparable in the absence (lane 3) or presence (lane 5) of MazF-mt3. Data shown are representative of two independent experiments. Complete gel images for (e–i) are shown inSupplementary Fig. 2. Figure 3: MazF-mt3 cleaves several M. tuberculosis mRNAs. Scale schematics of M. tuberculosis genes that contain either two or more MazF-mt3 UCCUU motifs ( a , b ), no MazF-mt3 motifs ( c ) or one UCCUU motif in the 5′ UTR but none in the ORF ( d ). Thin black arrows correspond to primers used for RT–PCR, while black lines with diamonds correspond to regions amplified by RT–PCR. Yellow arrows above genes show the location of UCCUU motifs. ( d ) Text above the schematic represents the RNA sequence of the senX3 5′ UTR (lowercase) and ORF (uppercase), with the lone MazF-mt3 motif in bold red text and a putative SD sequence in bold text. ( e – i ) RT–PCR of M. tuberculosis total RNA incubated with (lanes 5 and 6) or without (lanes 3 and 4) purified MazF-mt3 and with (lanes 3 and 5) or without reverse transcriptase (RT; lanes 1, 2, 4 and 6). ‘PCR +’ indicates amplification using the appropriate PCR fragment as a template (lane 1), while ‘C’ is a negative control with H 2 O as a PCR template (lane 2). Length of DNA size marker in bp is noted by tick marks on the right. After treatment with MazF-mt3, regions that contain one or more UCCUU motifs ( e , f , h ) no longer generated amplified products. This MazF-mt3-mediated cleavage was specific to regions containing one or more UCCUU motifs, since the amplified products in tuf ( g ) and in the senX3 ORF ( i ) were comparable in the absence (lane 3) or presence (lane 5) of MazF-mt3. Data shown are representative of two independent experiments. Complete gel images for ( e – i ) are shown in Supplementary Fig. 2 . Full size image MazF-mt3 targets critical components of the ribosome We also searched for cleavage sites within the E. coli transcriptome detected by MORE RNA-seq that are conserved in M. tuberculosis . From this analysis, we identified nine cleavage sites in E. coli genes that contain a MazF-mt3 recognition sequence within the same region of the orthologous gene in M. tuberculosis ( Supplementary Table 3 ). Among these nine cleavage sites, two were of significant interest because of their location within critical positions of 23S and 16S rRNA. In particular, MORE RNA-seq analysis identified a single MazF-mt3 cleavage site at 1940 U↓CCUU 1944 within helix/loop 70 of 23S rRNA ( Fig. 4 ) and at 1537 U↓CCUU 1541 within the aSD sequence at the 3′ end of 16S rRNA ( Fig. 5 ). These two cleavage sites are each located within a single-stranded region of both E. coli and M. tuberculosis rRNAs (according to the secondary structure of rRNAs from the Comparative RNA Web Site, http://www.rna.icmb.utexas.edu/ ) and are also the only UCCUU motifs in all rRNAs that are conserved between the two bacteria ( Supplementary Fig. 3 ). 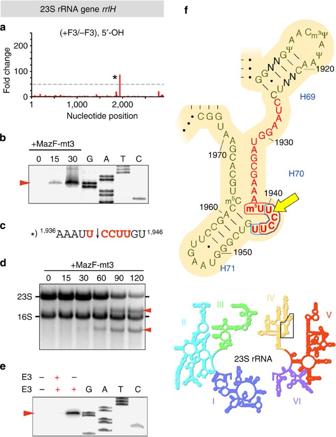Figure 4: MazF-mt3 cleaves 23S rRNA at a conserved UCCUU within helix/loop 70. (a) Histogram representing the ratio of #5′-ends observed in the analysis of 5′-OH from cells that did contain (+F3) or did not contain (−F3) MazF-mt3 within theE. coli23S rRNA generrlH. The lone cleavage site is labelled with an asterisk (*). (b) Primer extension analysis of 23S rRNA isolated fromE. colicells at the indicated time (0, 15 and 30 min) after the induction of MazF-mt3 expression. ‘G, A, T, C,’ sequencing ladder. The red arrow indicates the position of a cleavage product. (c) The RNA sequence surrounding the cleavage site (indicated by a black arrow) identified by MORE RNA-seq (a) and primer extension analysis (b), with flanking position numbers fromE. coli23S rRNA. (d) Ethidium bromide staining of total RNA isolated fromE. colicells at the indicated time (in min) after the induction of MazF-mt3 expression. (e) Primer extension analysis of 23S rRNA upon incubation of MazF-mt3 (F3) or MazE-mt3 (E3) withM. tuberculosistotal RNA. Complete gel images for (b,d,e) are shown inSupplementary Fig. 4. (f) Sequence and secondary structure of a conserved region of domain IV (above) in 23S rRNA (inset below). The nucleotides that comprise helix/loop 70 (H70) are highlighted in red text. Bases that are not conserved betweenE. coliandM. tuberculosisare labelled ‘N,’E. coliposition numbers are adjacent to tick marks, the MazF-mt3 recognition sequence is encircled by a blue line, the MazF-mt6 recognition sequence is encircled by a red line, and the site cleaved by both MazF-mt3 and MazF-mt6 is indicated by a yellow arrow. I–VI, numbered domains of 23S rRNA. Images in panel (f) are adapted from Yusupovet al.37and reprinted with permission from AAAS. Figure 4: MazF-mt3 cleaves 23S rRNA at a conserved UCCUU within helix/loop 70. ( a ) Histogram representing the ratio of #5′-ends observed in the analysis of 5′-OH from cells that did contain (+F3) or did not contain (−F3) MazF-mt3 within the E. coli 23S rRNA gene rrlH . The lone cleavage site is labelled with an asterisk (*). ( b ) Primer extension analysis of 23S rRNA isolated from E. coli cells at the indicated time (0, 15 and 30 min) after the induction of MazF-mt3 expression. ‘G, A, T, C,’ sequencing ladder. The red arrow indicates the position of a cleavage product. ( c ) The RNA sequence surrounding the cleavage site (indicated by a black arrow) identified by MORE RNA-seq ( a ) and primer extension analysis ( b ), with flanking position numbers from E. coli 23S rRNA. ( d ) Ethidium bromide staining of total RNA isolated from E. coli cells at the indicated time (in min) after the induction of MazF-mt3 expression. ( e ) Primer extension analysis of 23S rRNA upon incubation of MazF-mt3 (F3) or MazE-mt3 (E3) with M. tuberculosis total RNA. Complete gel images for ( b , d , e ) are shown in Supplementary Fig. 4 . ( f ) Sequence and secondary structure of a conserved region of domain IV (above) in 23S rRNA (inset below). The nucleotides that comprise helix/loop 70 (H70) are highlighted in red text. Bases that are not conserved between E. coli and M. tuberculosis are labelled ‘N,’ E. coli position numbers are adjacent to tick marks, the MazF-mt3 recognition sequence is encircled by a blue line, the MazF-mt6 recognition sequence is encircled by a red line, and the site cleaved by both MazF-mt3 and MazF-mt6 is indicated by a yellow arrow. I–VI, numbered domains of 23S rRNA. Images in panel ( f ) are adapted from Yusupov et al . [37] and reprinted with permission from AAAS. 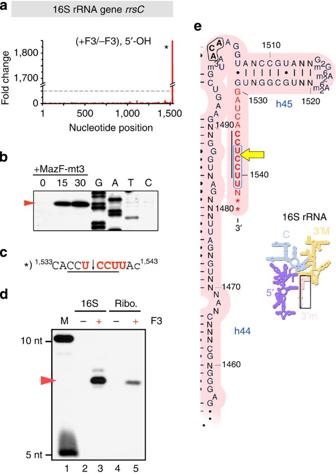Figure 5: MazF-mt3 cleaves within the aSD sequence, both in 16S rRNA and in ribosomes. (a) Histogram representing the ratio of #5′-ends observed in the analysis of 5′-OH from cells that did contain (+F3) or did not contain (−F3) MazF-mt3 within theE. coli16S rRNA generrsC. The lone cleavage site is labelled with an asterisk (*). (b) Primer extension analysis ofE. coli16S rRNA. (c) The RNA sequence surrounding the cleavage site identified by MORE RNA-seq (a) and primer extension analysis (b), with uppercase letters denoting nucleotides in the mature 16S rRNA and the final lowercase letter depicting the first nucleotide of the downstream intergenic region. (d) 3′-end-radiolabelledE. coli16S rRNA (16S) or 70S ribosomes (Ribo.) were incubated with (+) or without (−) purified MazF-mt3. The red arrow corresponds to a ~6-nt RNA fragment generated by MazF-mt3 cleavage. Marker lane (M) contains a mixture of 10-nt and 5-nt RNA oligonucleotides, each containing a 5′-end-radiolabel. Complete gel images for (b,d) are shown inSupplementary Fig. 5. (e) Secondary structure of a conserved region of the 3′ tail (above) of 16S rRNA (inset to the lower right). The 3′ tail, whose nucleotides are highlighted in red text, is identical betweenE. coliandM. tuberculosiswith the exception of two additional bases inM. tuberculosisat the very 3′ end, indicated with asterisks (*), and a single nonconserved base (N).E. coliposition number is adjacent to tick marks, theE. coliMazF recognition sequence (ACA) is in bold black text, the aSD sequence (CCUCCU) is in bold red text with a black line to the left, the MazF-mt3 recognition sequence (UCCUU) is in bold red text encircled by a blue line and the site cleaved by MazF-mt3 is indicated by a yellow arrow. 5′, 5′ domain of 16S rRNA; C, central domain; 3′M, 3′ major domain; and 3′m, 3′ minor domain; h44, helix 44; h45, helix 45. Images in panel (e) are adapted from Yusupovet al.37and reprinted with permission from AAAS. Full size image Figure 5: MazF-mt3 cleaves within the aSD sequence, both in 16S rRNA and in ribosomes. ( a ) Histogram representing the ratio of #5′-ends observed in the analysis of 5′-OH from cells that did contain (+F3) or did not contain (−F3) MazF-mt3 within the E. coli 16S rRNA gene rrsC . The lone cleavage site is labelled with an asterisk (*). ( b ) Primer extension analysis of E. coli 16S rRNA. ( c ) The RNA sequence surrounding the cleavage site identified by MORE RNA-seq ( a ) and primer extension analysis ( b ), with uppercase letters denoting nucleotides in the mature 16S rRNA and the final lowercase letter depicting the first nucleotide of the downstream intergenic region. ( d ) 3′-end-radiolabelled E. coli 16S rRNA (16S) or 70S ribosomes (Ribo.) were incubated with (+) or without (−) purified MazF-mt3. The red arrow corresponds to a ~6-nt RNA fragment generated by MazF-mt3 cleavage. Marker lane (M) contains a mixture of 10-nt and 5-nt RNA oligonucleotides, each containing a 5′-end-radiolabel. Complete gel images for ( b , d ) are shown in Supplementary Fig. 5 . ( e ) Secondary structure of a conserved region of the 3′ tail (above) of 16S rRNA (inset to the lower right). The 3′ tail, whose nucleotides are highlighted in red text, is identical between E. coli and M. tuberculosis with the exception of two additional bases in M. tuberculosis at the very 3′ end, indicated with asterisks (*), and a single nonconserved base (N). E. coli position number is adjacent to tick marks, the E. coli MazF recognition sequence (ACA) is in bold black text, the aSD sequence (CCUCCU) is in bold red text with a black line to the left, the MazF-mt3 recognition sequence (UCCUU) is in bold red text encircled by a blue line and the site cleaved by MazF-mt3 is indicated by a yellow arrow. 5′, 5′ domain of 16S rRNA; C, central domain; 3′M, 3′ major domain; and 3′m, 3′ minor domain; h44, helix 44; h45, helix 45. Images in panel ( e ) are adapted from Yusupov et al . [37] and reprinted with permission from AAAS. Full size image To validate the rRNA cleavage identified by MORE RNA-seq within helix/loop 70 of 23S rRNA ( Fig. 4a ), we first performed primer extension analysis of total RNA isolated from E. coli cells after the induction of MazF-mt3 ( Fig. 4b ). This analysis revealed a specific cleavage site at 1940 U↓CCUU 1944 of 23S rRNA ( Fig. 4c ; see schematic in Supplementary Fig. 3a ) that appeared within 15 min after MazF-mt3 induction and increased in abundance 30 min post induction ( Fig. 4b , Supplementary Fig. 4a ). We next analysed the effect of MazF-mt3 induction on 23S rRNA as visualized by staining total RNA with ethidium bromide ( Fig. 4d , Supplementary Fig. 4b ) and observed that the abundance of 23S rRNA was significantly reduced upon MazF-mt3 induction. Finally, we determined whether or not MazF-mt3 could cleave within helix/loop 70 of M. tuberculosis 23S rRNA. By use of primer extension analysis, we found that addition of purified MazF-mt3 to M. tuberculosis total RNA resulted in cleavage at 2178 U↓CCUU 2182 in helix/loop 70 of 23S rRNA ( Fig. 4e , Supplementary Fig. 4c ), a position analogous to the cleavage position in E. coli ( Supplementary Fig. 3a,c ). Thus, we conclude that MazF-mt3 targets helix/loop 70 of 23S rRNA. To validate the cleavage site identified by MORE RNA-seq within the aSD sequence of 16S rRNA ( Fig. 5a ), we also performed primer extension analysis of total RNA isolated from E. coli cells after the induction of MazF-mt3 ( Fig. 5b ). This analysis revealed a specific cleavage site at 1537 U↓CCUU 1541 of 16S rRNA ( Fig. 5c , see schematic in Supplementary Fig. 3b ) that appeared within 15 min after MazF-mt3 induction and increased in abundance 30 min post induction ( Fig. 5b , Supplementary Fig. 5a ). The cleavage of 16S RNA detected by MORE RNA-seq ( Fig. 5a ) and primer extension ( Fig. 5b ) occurs 5 nt from the 3′ end of mature 16S rRNA. Because MORE RNA-seq and primer extension analyses require the binding of a complementary oligonucleotide to a region several nucleotides downstream of a site of interest, these experiments must be detecting cleavage of 16S rRNA prior to its processing into a mature form. We therefore sought to establish whether or not MazF-mt3 could also cleave mature 16S rRNA. To do this, we incubated mature 16S rRNA containing a 3′-end radiolabel with MazF-mt3, separated the generated RNA fragments by gel electrophoresis and visualized radiolabelled RNA by autoradiography ( Fig. 5d and Supplementary Fig. 5b ). The results indicate that addition of MazF-mt3 to 16S rRNA generated a small RNA fragment ~6 nt in length, consistent with cleavage at 1537 U↓CCUU 1541 of 16S rRNA. We conclude that MazF-mt3 can cleave both the precursor ( Fig. 5a,b ) and mature forms ( Fig. 5d and Supplementary Fig. 5b , lane 3) of 16S rRNA. We next tested whether MazF-mt3 could cleave 16S rRNA in the context of the ribosome. To do this, we introduced a 3′ end radiolabel to rRNA in 70S ribosomes. Addition of MazF-mt3 to 70S ribosomes generated the same small RNA fragment ~6 nt in length that appeared in reactions with 16S rRNA alone ( Fig. 5d and Supplementary Fig. 5b , compare lanes 3 and 5). We conclude that MazF-mt3 can cleave at 1537 U↓CCUU 1541 at the aSD sequence of 16S rRNA within the context of 70S ribosomes. Here we describe a high-throughput approach, MORE (mapping by overexpression of an RNase in E. coli ) RNA-seq ( Fig. 1 ), which facilitates determination of the cleavage specificity of endoribonucleolytic toxins and is broadly applicable to any single-strand-specific endoribonuclease. As demonstrated by our analysis of Maz-mt3 ( Fig. 2 ), the positive attributes of MORE RNA-seq supersede the full complement of conventional approaches. In particular, MORE RNA-seq allowed us to pinpoint an unambiguous cleavage recognition sequence, precisely map the position of cleavage within this sequence and reveal whether the ends generated upon cleavage carry a 5′-OH or a 5′-P. In addition, our MORE RNA-seq analysis of MazF-mt3 provides a foundation towards understanding the role of this toxin in M. tuberculosis by enabling comprehensive identification of putative target RNAs, including UCCUU-containing transcripts ( Fig. 3 and Supplementary Tables 2–4 ) and two critical rRNA sites ( Figs 4 and 5 ). There are numerous advantages of MORE RNA-seq over conventional approaches for cleavage consensus determination. First, when used for RNA-cleaving TA toxins, MORE RNA-seq accurately identifies a complete, unambiguous cleavage recognition sequence. In contrast, use of conventional approaches routinely identifies degenerate or inaccurate consensus sequences [14] , [17] , [18] , [20] , [21] , [27] , [28] , [29] . For example, the cleavage consensus sequence for MazF-mt3 had previously been determined using a conventional primer extension-based approach and was reported as CU↓CCU or UU↓CCU on the basis of an alignment of 12 cleavage sites from a single RNA substrate [20] . Our MORE RNA-seq analysis of MazF-mt3 identified the recognition sequence as U↓CCUU ( Fig. 2c ) after alignment of 273 cleavage sites ( Supplementary Data 1 ). We suspect that in the prior study, the limited length and unequal cleavage motif representation of the substrate RNA coupled with in vitro reaction conditions in which the toxin was in molar excess of the substrate account for the identification of a degenerate sequence. In contrast, MORE RNA-seq exploits the unparalleled depth of the entire E. coli transcriptome and enables cleavage to occur in living cells. Second, the base-pair resolution of MORE RNA-seq enables one to precisely pinpoint the position of cleavage and overcome the inherent ambiguity associated with data obtained by conventional approaches. When analysed by primer extension or by cleavage of synthetic RNA substrates, RNA-cleaving TA toxins are routinely reported to exhibit cleavage on either side of a base or at multiple positions within a given recognition sequence [6] , [7] , [17] , [21] , [23] , [24] , [25] , [27] , [29] . For example, E. coli MazF is proposed to cut both before and after the first A of its recognition sequence (↓ACA or A↓CA) [6] . Our results demonstrated that MazF-mt3 cleaves with high precision after the first U of the U↓CCUU consensus sequence ( Fig. 2c , Supplementary Data 1 ). Thus, we propose that cleavage of RNA by TA toxins within their respective recognition sequences is invariant and that reports of ambiguous positions of cleavage are a byproduct of the intrinsic limitations of the methods used for their identification. Third, because MORE RNA-seq is a genome-scale approach, it enables the identification of relatively long cleavage recognition sequences. While E. coli MazF cleaves RNA at a 3-base recognition sequence, many MazF toxins require more complex sequences [14] , [15] , [16] , [19] , [20] , [23] , [24] , [25] , [26] . Although it was extremely difficult to deduce, the longest MazF recognition sequence reported to date is 7 nt [16] . Thus, to identify a cleavage consensus sequence greater than 5 nt, the full complement of traditional approaches are, at best, extremely time-intensive [16] and, at worst, may fail if the recognition sequence is underrepresented in the substrate RNAs that are analysed. Assuming an equal base content, equal representation of all potential cleavage motifs, and no secondary structure, one would need to survey 4 6 or 4,096 nt of RNA to identify just one cleavage site with a single 6-base recognition sequence, and 16,384 nt for a 7-base sequence. Since many cleavage sites are needed to deduce an unambiguous consensus sequence, the overall substrate length needed to determine the cleavage specificity of toxins with relatively long recognition sequences is simply not attainable using only highly expressed transcripts or in vitro templates. Fourth, MORE RNA-seq can identify cleavage sites in regions that would typically be overlooked by conventional approaches, such as those in 5′ and 3′ UTRs, intergenic regions, or non-coding transcripts like tRNAs, rRNAs and antisense and small RNAs. In particular, tRNAs and rRNAs are routinely overlooked due to extensive secondary structure that makes them difficult and unattractive templates for primer extension, while other non-coding RNAs are overlooked by traditional methods since only highly abundant transcripts can be easily interrogated. However, MORE RNA-seq readily detects cleavage sites regardless of their position in coding or non-coding RNA, since 22% (60 of 273) of the sites we identified in our analysis of MazF-mt3 are in non-coding regions ( Supplementary Data 1 ). In addition, we demonstrated that a MazF-mt3 cleavage event occurs 5 nt from the 3′ end of mature 16S rRNA. Cleavage at this position would be undetectable by northern analysis or primer extension analysis of mature 16S rRNA. Thus, the exquisite sensitivity of MORE RNA-seq uncovered an unexpected role for a M. tuberculosis MazF toxin and suggests there may be some functional parallels between how MazF toxins enlist 16S rRNA to influence cell physiology. Finally, MORE RNA-seq can readily determine the cleavage specificity of toxins from intractable prokaryotes. Elucidating the physiological roles of TA systems in the context of extremophilic, fastidious or pathogenic organisms is challenging due to the inherent limitations of organisms that are often genetically intractable or require specialized conditions to grow in the laboratory. For example, M. tuberculosis , which has an overwhelming abundance of TA systems, is slow growing (doubling every 24 h), requires BSL3 containment, and lacks experimental tools for detailed molecular manipulation. An essential first step in defining the physiological targets of toxins or endonucleases that cleave RNA is to determine their cleavage specificities. MORE RNA-seq thus provides a useful methodology to define cleavage specificities of endoribonucleases from organisms that are not easily amenable to laboratory manipulation because this method is carried out in E. coli , a BSL1 organism that is genetically tractable and rapidly growing. In addition, the use of E. coli as a platform to identify cleavage sites enables a given toxin or endonuclease to be interrogated within the context of a living cell that lacks a 5′-to-3′ exonucleolytic activity, unlike many of the organisms that carry endoribonucleolytic toxins. Toxins in the MazF family have been labelled ‘mRNA interferases’ because they cleave mRNA and because they initially did not appear to cleave tRNAs or rRNAs [7] , [8] , [12] , [13] , [16] , [17] . However, this view has been challenged by two recent studies showing that MazF toxins can, in fact, target rRNA. First, Vesper et al. [22] demonstrated that E. coli MazF cleaves at a single site near the 3′ end of 16S rRNA in vivo ( Fig. 5e ), resulting in the loss of the terminal 43 nt including the aSD sequence. Ribosomes containing this truncated 16S rRNA (‘stress ribosomes’) exhibit a preference for leaderless mRNAs that are either naturally present in the cell or generated by MazF cleavage [22] , [32] . Second, Schifano et al. [23] showed that M. tuberculosis toxin MazF-mt6 inactivates the ribosome by cleaving helix/loop 70 in 23S rRNA ( Fig. 4f ). Strikingly, we find that MazF-mt3 targets the same functional regions of 23S and 16S rRNA that are targeted by MazF-mt6 and E. coli MazF, respectively. In particular, MazF-mt3 cleaves 23S rRNA at the exact position within helix/loop 70 in 23S rRNA as MazF-mt6 ( Fig. 4f ). In addition, MazF-mt3 cleaves near the 3′ end of 16S rRNA to remove the aSD sequence ( Fig. 5e ). Thus, in spite of recognizing a sequence (U↓CCUU) that is distinct from that of MazF-mt6 (UU↓CCU) and E. coli MazF (↓ACA), MazF-mt3 targets the same functional regions of rRNA as these other MazF toxins. MazF-mt3 cleavage of 23S rRNA is projected to have a significant impact on cellular translation since helix/loop 70 ( Fig. 4f ) is essential for ribosome function due to its location in the ribosomal A site and its stabilization of tRNA and ribosome recycling factor [33] , [34] , [35] , [36] , [37] . In fact, cleavage at this site by toxin MazF-mt6 is sufficient to disable translation [23] . However, the significance of MazF-mt3-mediated cleavage of the aSD sequence in 16S rRNA ( Fig. 5 ) and the potential role of MazF-mt3-truncated ribosomes in translating leaderless mRNAs ( Fig. 3h ) are less clear. The M. tuberculosis genome encodes very few genes—only nine—with MazF-mt3 UCCUU motifs upstream of the start codon from which leaderless mRNAs can be generated, and only seven of these do not have a UCCUU motif elsewhere in the ORF ( Supplementary Table 4 ). We tested one of these seven, senX3 , that encodes an essential two-component sensor histidine kinase associated with virulence [38] . As predicted, MazF-mt3 cleaved within the senX3 5′ UTR to generate a leaderless transcript ( Fig 3d,h ). Although there is a relative dearth of these potential MazF-mt3-generated leaderless transcripts, this may be offset by the unusual abundance (26%) of naturally leaderless mRNAs in M. tuberculosis cells [39] . Since we have demonstrated that MazF-mt3 can indeed cleave the aSD sequence from 16S rRNA within ribosomes ( Fig. 5d ), it is possible that the affected ribosomes may also exhibit specificity for leaderless mRNAs in a manner similar to those created in E. coli by MazF. The overall dynamic of MazF action in E. coli is much different than that predicted for MazF-mt3 in M. tuberculosis. In E. coli , 99% of mRNAs (4,192 of 4,243) are susceptible to MazF cleavage [12] , so widespread mRNA degradation likely occurs in conjunction with the production of ‘stress ribosomes.’ In contrast, only 20% of mRNAs (807 of 4,022) in M. tuberculosis contain one or more UCCUU MazF-mt3 cleavage sequences, suggesting mRNA cleavage is not as prevalent with this toxin. In addition, the two distinct rRNA sites targeted by MazF-mt3 appear to differentially impact cellular translation. Cleavage at helix/loop 70 of 23S rRNA disables translation [23] , while removal of the aSD sequence is likely not as severe, since the loss of helix 45 and the aSD-containing 3′ tail only precludes recognition of Shine-Dalgarno (SD) sequences in canonical mRNAs by affected ribosomes [22] . Not only it is unknown what phenotype would result from SD-independent translation in M. tuberculosis , but several reports document the dispensability of the aSD sequence for selecting the correct translation start site [40] , [41] , [42] . Therefore, MazF-mt3 may possess dual functionality, with the potential to either completely inactivate the ribosome via 23S rRNA cleavage or alter the specificity of the ribosome by removing the aSD sequence. It is unknown to what degree 23S and 16S rRNA in M. tuberculosis are cleaved by MazF-mt3 in vivo , but it is intriguing to speculate that these rRNAs are differentially susceptible to cleavage and that distinct phenotypes might arise from preferential cleavage of either rRNA. Finally, we find that distinct MazF toxins target the same regions of rRNA. Given that a significant portion of rRNA is likely refractory to the action of single-strand-specific endoribonucleases, we propose that certain MazF toxins have evolved recognition specificities that enable them to exploit essential and accessible regions within the translation machinery as a means of causing efficient growth inhibition. Accordingly, we propose that helix/loop 70 in 23S rRNA and the aSD sequence in 16S rRNA constitute an ‘Achilles heel’ of the translational apparatus. It remains to be determined whether other regions of rRNA will also emerge as common targets of endoribonucleolytic toxins. If other vulnerable regions exist in rRNA, MORE RNA-seq provides a useful means of facilitating their discovery. Strains, plasmids and reagents The E. coli strains BW25113Δ6 [ lacI q rrnB T14 Δ lac-Z WJ16 hsdR514 Δ araBAD AH33 Δ rhaBAD LD78 Δ chpBIK Δ dinJ-yafQ Δ hipBA Δ mazEF Δ relBE Δ yefM-yoeB ] [43] and BL21(DE3) [F − omp T hsd S β (r β − , m β − ) dcm gal λ(DE3); Novagen] were used for all RNA cleavage/growth profile and protein expression studies, respectively. E. coli Mach1-T1 [F – Δ rec A1398 end A1 ton A ϕ80( lacZ) ΔM15 Δ lac X74 hsd R(r κ − , m κ + ); Invitrogen] cells were used for all cloning experiments. Plasmids used in this study include pBAD33 (ref. 44 ), pIN-III (ref. 45 ) and pET-21c and pET-28a (Novagen). The mazF-mt3 gene ( Rv1991c locus) was PCR-amplified from M. tuberculosis strain H37Rv genomic DNA with 5′-NdeI/BamHI-3′ ends to create pET-28a- mazF-mt3 (ref. 20 ) and pET-21c- mazF-mt3 . To create pBAD33- mazF-mt3 , the pET-21c- mazF-mt3 plasmid was digested with XbaI and HindIII to include the highly efficient T7 phage ribosome binding site, and the resulting fragment was cloned into pBAD33 (ref. 21 ). The mazE-mt3 gene ( Rv1991A locus) was PCR-amplified from M. tuberculosis strain H37Rv genomic DNA with 5′-NdeI/BamHI-3′ ends to create pET-28a- mazE-mt3 (ref. 46 ) and pIN-III- mazE-mt3 . To generate sequencing ladders for primer extension analysis, E. coli 23S and 16S rRNA genes were PCR-amplified from E. coli strain BW25113Δ6 cultures and ligated into Strataclone PCR cloning vectors (Agilent) to create pSC-A-Eco23S and pSC-A-Eco16S, respectively. Mycobacterial 23S rRNA was PCR-amplified from Mycobacterium smegmatis strain mc 2 155 genomic DNA and ligated into a Strataclone PCR cloning vector (Agilent) to create pSC-A-Myco23S, which was used to create sequencing ladders for M. tuberculosis , since the sequence of M. smegmatis and M. tuberculosis 23S rRNAs are 100% identical for a >160-nt region upstream of the NWO1571 primer used. Clones were confirmed by DNA sequence analysis. All E. coli liquid cultures were grown at 37 °C in M9 minimal medium supplemented with casamino acids to a final concentration of 0.2% and either glucose to a concentration of 0.2% or glycerol to 0.1%. The toxin was expressed from an arabinose-inducible promoter in pBAD33- mazF-mt3 , while the antitoxin was expressed from an isopropyl-β- D -thiogalactopyranoside (IPTG)-inducible promoter in pIN-III- mazE-mt3 . The working concentrations of kanamycin, ampicillin and chloramphenicol were 50, 100 and 25 μg ml −1 , respectively. RNA isolation for MORE RNA-seq Total RNA was isolated from E. coli strain BW25113Δ6 harbouring either pBAD33 or pBAD33- mazF-mt3 grown to mid-logarithmic phase. When cultures reached an OD 600nm of 0.4, arabinose was added to a final concentration of 0.2%, and growth continued for an additional 15, 30, 60, 90 or 120 min post induction. Cells were pelleted by centrifugation at 2,000 g for 10 min, and supernatants were removed. Cell pellets were resuspended in TRIzol Reagent (Invitrogen) and lysed for 10 min at 60 °C. Lysates were extracted with chloroform and precipitated with ethanol according to the TRIzol Reagent protocol. RNA pellets were dissolved in nuclease-free water, treated with TURBO DNase (Invitrogen) for 45 min at 37 °C, extracted with acid phenol chloroform and precipitated with ethanol. Preparation of RNA for high-throughput sequencing The general procedure to prepare RNA for high-throughput sequencing was essentially as described in Goldman et al. [47] with some modifications similar to Vvedenskaya et al. [48] as follows. Two major alterations were designed with a goal of retaining small RNA cleavage fragments and potentially obtaining cleavage sites in rRNA. To this end, total RNA was not passed through an RNeasy Mini Kit (Qiagen) to remove RNA less than ~200 nt, and rRNAs were not depleted. Total RNA harvested 15 min post induction was used. Two major RNA pools were isolated, one with 5′-P ends and one with 5′-OH. To isolate RNAs with a 5′-P, 1 μg RNA was ligated directly to the 5′ SOLiD RNA adaptor (5′-CCACUACGCCUCCGCUUUCCUCUCUAUGGGCAGUCGGUGAU-3′). To isolate RNAs with a 5′-OH, 2 μg RNA was treated with 1 U of Terminator 5′-Phosphate-Dependent Exonuclease (Epicentre) to remove RNAs with a 5′-P, followed by phosphorylation by 50 U of OptiKinase (Affymetrix) to convert 5′-OH to 5′-P suitable for ligation. The resultant RNAs with a 5′-P were then ligated to the 5′ adaptor. Ligation reactions contained 5′-P RNA, 75 pmol 5′ SOLiD adaptor, and 20 U T4 RNA Ligase I (New England Biolabs). Ligations were incubated for 2 h at 37 °C and then for 14 h at 16 °C. Ligation reactions were electrophoresed on a 6% (wt/vol) polyacrylamide 7 M urea gel in TBE buffer, and RNAs that migrated above the free 5′ adaptor were isolated by gel excision. After ligation, cDNAs were generated by reverse transcription using a primer that contained nine degenerate nucleotides at the 3′ end and a common ‘3′ SOLiD adaptor’ sequence (5′-CTGCTGTACGGCCAAGGCGNNNNNNNNN-3′). The annealing step was performed by first mixing 150–400 ng of 5′ adaptor-ligated RNA with 30 pmol of the RT primer and incubating for 3 min at 85 °C to allow unfolding of extensive secondary structures in rRNAs followed by 5 min at 4 °C. Reverse transcription was performed by adding a cocktail containing 200 U SuperScript III reverse transcriptase (Invitrogen), reaction buffer, dNTPs and RNase inhibitor (RNaseOUT (Invitrogen)) to the RT primer-RNA mixture and incubated first for 5 min at 25 °C, then 60 min at 55 °C. The reverse transcriptase was then inactivated by incubating for 15 min at 70 °C. Next, to remove the RNA strand from the RNA–DNA hybrids, 10 U of RNase H (Ambion) was added, and reactions were incubated for 20 min at 37 °C. The samples were then electrophoresed on a 10% (wt/vol) polyacrylamide 7 M urea gel, and cDNAs that migrated between ~125 nt and ~500 nt were isolated after gel excision. PCR of cDNA was performed with an initial denaturation step of 30 s at 98 °C, amplification for 14 cycles (denaturation for 10 s at 98 °C, annealing for 20 s at 62 °C and extension for 10 s at 72 °C), and a final extension for 7 min at 72 °C using reagents from a SOLiD total RNA-seq kit and primers from a SOLiD RNA barcoding kit (Applied Biosystems). After electrophoresis on a non-denaturing 10% (wt/vol) polyacrylamide gel, amplified DNA that migrated between the positions of the 150 bp and 300 bp DNA standards was isolated after gel excision and sequenced using an Applied Biosystems SOLiD system, version 4.0. Identification of MazF-mt3 cleavage sites by MORE RNA-seq Sequencing reads for which the first 30 bases mapped with 0 mismatches to the E. coli MG1655 genome were identified using Bowtie (version 1.0.0) [49] . For each position in the genome, the number of sequencing reads whose first base aligned to that position was calculated (this value we refer to as #5′-ends). Next, we added a pseudocount to the genomic positions for which the #5′-ends was 0. We then divided the #5′-ends from the analysis of RNA isolated from cells containing MazF-mt3 by the #5′-ends from cells that did not contain MazF-mt3. We identified genomic positions for which this ratio was ≥50 in the analysis of both biological replicates. In addition, we required that the position of enrichment represented local maxima within a 20 base window spanning 10 bases up- and downstream. In the analysis of RNAs carrying a 5′-OH, we identified 273 positions that met these criteria ( Supplementary Data 1 ), while in the analysis of RNAs carrying a 5′-P, we identified only two positions. For cleavage sites that mapped to more than one position in the genome due to redundant sequences, each position and locus were noted in Supplementary Data 1 ; the sequence surrounding the cleavage site was only counted once to determine the consensus sequence in Fig. 2c . Preparation of recombinant His 6 -MazF-mt3 and His 6 -MazE-mt3 pET-28a- mazF-mt3 and pET-28a- mazE-mt3 BL21(DE3) transformants were used to inoculate 1 l of M9 liquid medium (supplemented with 0.2% casamino acids) and grown to an OD 600nm of 0.6. Transformants were induced with a final concentration of 1 mM IPTG and expressed for 2.5 h. Cells were disrupted by sonication, and extracts were purified by nickel–nitrilotriacetic acid affinity chromatography (Qiagen). RT–PCR of M. tuberculosis total RNA incubated with MazF-mt3 Total RNA was isolated from M. tuberculosis strain H37Rv grown to mid-logarithmic phase. Cell pellets were resuspended in TRIzol Reagent (Ambion). Lysates were extracted with chloroform and precipitated with ethanol according to the supplier’s protocol. RNA pellets were dissolved in nuclease-free water, treated with 10 U of DNase I (Invitrogen) for 60 min at 37 °C, extracted with acid phenol chloroform and precipitated with ethanol. DNase-treated RNA (11.7 μg) was incubated for 30 min at 37 °C in 10 mM Tris-HCl with 7 U of RNase inhibitor (New England Biolabs) and either with or without 139 pmol of purified MazF-mt3 to a final concentration of 1 μM. RNA was extracted twice with phenol–chloroform–isoamyl alcohol and precipitated with ethanol. Reverse transcription was performed using the SuperScript III First-Strand Synthesis System (Invitrogen) with the following slight modifications to the supplier’s protocol. The annealing step was performed with 1 μg of either MazF-mt3-treated or -untreated RNA and 30 ng of random hexamer primers for 5 min at 65 °C, followed by 1 min at 4 °C. The reverse transcription step was performed in a 20 μl reaction with the primer-RNA mixture, 200 U of SuperScript III reverse transcriptase and 40 U of RNaseOut by incubating first for 5 min at 25 °C, then 20 min at 52.5 °C. The reverse transcriptase was then inactivated by incubating for 5 min at 85 °C. PCR of the resulting cDNA (or genomic M. tuberculosis DNA as a positive control or H 2 O as a negative control) was performed with an initial denaturation step of 3 min at 94 °C, amplification for either 26 cycles for senX3 or 27 cycles for the Rv1685c , Rv1545 and tuf genes (denaturation for 45 s at 94 °C, annealing for 30 sec at 53 °C, and extension for 15 s at 72 °C) and a final extension for 5 min at 72 °C. Amplicon sizes and PCR primers were as follows: Rv1685c 156-bp, forward (Fwd; 5′-GTCGAGGAACTCGGTTACAAGCTGC-3′) and reverse (Rev; 5′-AAGCTCCACGGTGACCACTTCC-3′); Rv1545 150-bp, Fwd (5′-CAGTGCTGCCAGATGCACAAT-3′) and Rev (5′-CTAAGGAGCGGCGCCATC-3′); tuf 151-bp, Fwd (5′-ACGTCTTCACCATTACCGGC-3′) and Rev (5′-AGCAGCTTGCGGAACATCTC-3′); senX3 5′ UTR 153-bp, Fwd (5′-CGTAGTGTGTGACTTGTCCGATTTTGGC-3′) and Rev (5′-GCATTCCAACAGCACCACCGAC-3′); and senX3 ORF 165-bp, Fwd (5′-GCGGCTACCCAATATGACCG-3′) and Rev (5′-TTTGCCAGTGCGGTAACCAG-3′). The reactions were run on a 2% (wt/vol) agarose gel and visualized by staining with ethidium bromide. In vivo primer extension analysis Total RNA from E. coli expressing MazF-mt3 (25 μg) was used in primer extension reactions, and sequencing ladders were generated by using plasmids carrying E. coli rRNA genes (pSC-A-Eco23S or pSC-A-Eco16S) and a Sequenase version 2.0 DNA sequencing kit (Affymetrix) according to the Sequenase kit protocol, both essentially as described in Sharp et al. [50] . DNA oligonucleotides were radiolabelled at the 5′ end by treating with T4 polynucleotide kinase (New England Biolabs) and [γ- 32 P]ATP (PerkinElmer) for 1 h at 37 °C. The oligonucleotide NWO1556 (5′-CACTGCATCTTCACAGCGAGTTCAATTTC-3′) was used for 23S rRNA, and the primer NWO1983 (5′-CGCCTTGCTTTTCACTTTTCATCAGACAATC-3′) was used for 16S rRNA. Primer NWO1983 is located in the intergenic region downstream of mature 16S rRNA and was designed to detect all seven rRNA loci in E. coli by selecting the most conserved nucleotide at each position. Cleavage products were detected by extending 0.7 pmol of gene-specific 5′-end-radiolabelled oligonucleotides with 5 U of avian myeloblastosis virus reverse transcriptase (New England Biolabs) in a 20-μL reaction volume for 1 h at 53 °C. All reactions were electrophoresed on a 6% (wt/vol) polyacrylamide 7 M urea gel and visualized by autoradiography. In vitro primer extension analysis of M. tuberculosis total RNA Total RNA from M. tuberculosis strain H37Rv (4.0 μg) was used, and primer extension analysis was performed essentially as described in Schifano et al. [23] . For antitoxin inhibition of RNA cleavage, MazE-mt3 was preincubated with MazF-mt3 for 10 min at room temperature before the RNA substrate was added. RNA was incubated with or without a final concentration of 1.0 μM MazF-mt3 or 2.0 μM MazE-mt3 in 10 mM Tris-HCl (pH 7.8) for 15 min at 37 °C. For primer extension, the reaction components, amounts and conditions were the same as described above for in vivo primer extension analysis. The oligonucleotide NWO1571 (5′-CGAGCATCTTTACTCGTAGTGCAATTTCG-3′) was used for both primer extension and sequencing reactions. Sequencing ladders were generated as described above except pSC-A-Myco23S was used as a template. Reactions were electrophoresed as described above. Treatment of E. coli 16S rRNA or ribosomes with MazF-mt3 in vitro 16S rRNA was isolated from E. coli total RNA by excising the appropriate part of the gel after electrophoresis in denaturing formaldehyde agarose, while E. coli 70S ribosomes were purchased (New England Biolabs). The rRNAs were radiolabelled at the 3′ end using E. coli poly(A) polymerase (New England Biolabs), 1 × E. coli poly(A) polymerase reaction buffer, and [α- 32 P]ATP (PerkinElmer). To discourage the addition of multiple adenine residues, we used submolar amounts of [α- 32 P]ATP relative to the RNA substrate—either an [α- 32 P]ATP:RNA ratio of 1:30 for 16S rRNA or a ratio of 1:15 for ribosomes—similar to a study by Martin and Keller [51] . The radiolabelling reaction was incubated for 1.5 h at 37 °C and stopped by the addition of EDTA to a final concentration of 10 mM to sequester Mg 2+ ions and inhibit E. coli poly(A) polymerase. The radiolabelled 16S rRNA or ribosomes (0.05 μM final concentration) were supplemented with magnesium acetate to a final concentration of 10 mM and incubated either with purified MazF-mt3 to a 1.0 μM final concentration or with no toxin for 1 h at 37 °C. Cleavage reactions were stopped by the addition of either loading dye with formamide for 16S rRNA or phenol–chloroform–isoamyl alcohol for ribosomes. Ribosome reactions were extracted twice with phenol–chloroform–isoamyl alcohol and precipitated with ethanol. All cleavage reactions were electrophoresed on a 22.5% (wt/vol) polyacrylamide 7 M urea gel in TBE buffer and visualized by autoradiography. To estimate the size of cleaved fragments, 10-nt (5′-AUCCGGAAUC-3′) and 5-nt (5′-CGCCU-3′) RNA oligonucleotides were radiolabelled at the 5′ end by treating with T4 polynucleotide kinase (New England Biolabs) and [γ- 32 P]ATP (PerkinElmer) for 1 h at 37 °C. Reversible inhibition of growth by mazEF-mt3 expression MazF-mt3 was expressed ectopically in E. coli strain BW25113Δ6 liquid cultures from an arabinose-inducible promoter in pBAD33- mazF-mt3 , while MazE-mt3 was expressed from an IPTG-inducible promoter in pIN-III- mazE-mt3 . To discourage leaky expression of MazF-mt3, glucose was added to M9 liquid medium (supplemented with 0.2% casamino acids) to a final concentration of 0.2% at all times until immediately before induction of the toxin. E. coli double transformants harbouring either pBAD33- mazF-mt3 +pIN-III or pBAD33- mazF-mt3 +pIN-III- mazE-mt3, were grown overnight and diluted to an OD 600nm of 0.06. Cultures were grown at 37 °C to an OD 600nm of 0.27 (1 h post dilution), centrifuged at 3,200 g for 5 min, resuspended in M9 liquid medium with 0.1% glycerol and arabinose was added to both cultures to a final concentration of 0.05% to induce MazF-mt3. After 60 min of growth inhibition (2 h post dilution), IPTG was added to both cultures to a final concentration of 1 mM to either induce MazE-mt3 or serve as a control. Analysis of UCCUU frequency in M. tuberculosis genes All 4,095 annotated non-coding RNA and protein-coding genes from M. tuberculosis strain H37RV were retrieved from the TubercuList Web site ( http://www.tuberculist.epfl.ch/ ) on 17 August 2012. These genes were divided into 11 functional categories from the genome annotation [52] , [53] , [54] . Six loci— Rv0298 , Rv0299 , Rv0909 , Rv0910 , Rv2653c and Rv2654c —that Cox and coworkers found to be novel functional TA systems [11] were moved into the ‘virulence, detoxification and adaptation’ category. The Rv2653c and Rv2654c loci were removed from the ‘insertion sequences and phages’ group, while the other four genes were removed from the ‘conserved hypothetical protein’ category. The nucleotide composition of each gene was calculated. The probability, p , of the MazF-mt3 cleavage motif UCCUU appearing anywhere in an M. tuberculosis gene is p =(percentage of U) [3] × (percentage of C) [2] . Let L be the length of the gene. Then the expected number, E , of motifs in the gene is E = p ( L− 4). Let K be the actual number of motifs in the gene. Then the probability, P , of having K or more motifs in the gene is: A gene with a very small P -value may have evolved to be susceptible to cleavage by MazF-mt3. Accession codes : The RNA sequencing data have been deposited in the NCBI Sequence Read Archive under accession code SRP037999 . How to cite this article : Schifano, J. M. et al. An RNA-seq method for defining endoribonuclease cleavage specificity identifies dual rRNA substrates for toxin MazF-mt3. Nat. Commun. 5:3538 doi: 10.1038/ncomms4538 (2014).